Lifespan maturation and degeneration of human brain white matter Properties of human brain tissue change across the lifespan. Here we model these changes in the living human brain by combining quantitative magnetic resonance imaging (MRI) measurements of R1 (1/ T 1) with diffusion MRI and tractography ( N =102, ages 7–85). The amount of R 1 change during development differs between white-matter fascicles, but in each fascicle the rate of development and decline are mirror-symmetric; the rate of R 1 development as the brain approaches maturity predicts the rate of R 1 degeneration in aging. Quantitative measurements of macromolecule tissue volume (MTV) confirm that R 1 is an accurate index of the growth of new brain tissue. In contrast to R 1, diffusion development follows an asymmetric time-course with rapid childhood changes but a slow rate of decline in old age. Together, the time-courses of R 1 and diffusion changes demonstrate that multiple biological processes drive changes in white-matter tissue properties over the lifespan. Over the past decade, it has become clear that white matter plays a critical role in nearly every aspect of cognitive development, healthy cognitive function and cognitive decline in aging. Moreover, many psychiatric disorders—from autism to schizophrenia—are associated with white-matter abnormalities [1] , [2] . White-matter tissue properties change over the lifespan and models of the biological principles underlying these changes are critical for understanding the process of brain maturation and for diagnosing abnormalities in the living human brain. Advances in quantitative magnetic resonance imaging (qMRI) now make it possible to measure and model the biological properties of tissue in the living human brain. Each qMRI parameter is sensitive to different properties of the tissue [3] , [4] , [5] , [6] , [7] , [8] , [9] , [10] , [11] . By combining the information from different types of qMRI measurements and known biophysical properties of different tissue types, it is possible to reason about changes in the biological composition of the tissue over the lifespan. To date, most qMRI investigations of lifespan changes in white-matter tissue structure have focused on diffusion-weighted magnetic resonance imaging (dMRI). Due to improvements in dMRI acquisitions and software, spatially resolved measurements of specific white-matter fascicles or tracts are now routine and there is a substantial literature documenting changes in white-matter diffusion properties over the lifespan [12] , [13] , [14] , [15] , [16] , [17] . From these measurements, retrogenesis has emerged as a widely discussed principle of brain development and aging [18] , [19] , [20] , [21] . Retrogenesis postulates that late maturing tissue is particularly vulnerable during aging and that tissue degeneration in the aging brain follows the reverse sequence of tissue maturation in the developing brain. This theory conceptualizes brain development like building a pyramid where the base is stabilized before additional layers are added. The top of the pyramid is the most vulnerable to aging-related decline, while the base remains sturdy. Retrogenesis has not been formalized in a manner that makes specific quantitative predictions, and several distinct hypotheses are discussed under the principle of retrogenesis [17] , [21] , [23] . White matter is composed of many different types of tissue including myelin, astrocytes, microglia and oligodendrocytes, and each tissue type might change with its own unique time-course [14] , [24] . For example, myelinated axons might change in a manner that is consistent with the retrogenesis hypothesis, while glial tissue might not. Diffusion measurements are open to many biological interpretations [9] , [25] , [26] , and there may be multiple, independent, biological processes active across the lifespan that cannot be separated with diffusion measurements alone. R 1 (1/ T 1), a measure of the longitudinal relaxation rate of water hydrogen protons in a magnetic field, provides complementary information to measures of diffusion properties. In white matter, R 1 is primarily driven by variation in myelin content (~90%; ref. 27 ). The significance of R 1 for biological measurements has been recognized for decades [6] , [28] , [29] , but fast, accurate and reliable measurement methods have only recently become available [7] , [30] , [31] . Here we employ a novel quantitative R 1 mapping procedure [7] in combination with dMRI and tractography to model the processes underlying changes in white-matter tissue composition that occur between childhood and old age. Combining multiple measurement modalities makes it possible to dissociate multiple biological processes that progress independently over the lifespan. Consistent with the retrogenesis hypothesis, in each fascicle the rate of R 1 development as the brain approaches maturity closely matches the rate of R 1 degeneration in aging. Measurements of macromolecule tissue volume (MTV) confirm that R 1 is an accurate index of tissue creation and loss. Unlike R 1, diffusivity changes follow an asymmetric time-course, revealing a second lifespan process that does not follow the principle of retrogensis. Finally, we show that these quantitative lifespan models of white-matter tissue changes can be used to detect and quantify degeneration of specific fascicles in individual patients with degenerative disorders of the white matter (multiple sclerosis (MS)). Models of the processes underlying healthy white-matter maturation will offer new insight into the coupling between biological and cognitive development and allow white-matter abnormalities to be rapidly diagnosed and monitored. White-matter tissue properties change in relation to age We modelled changes in R 1 relaxation (1/ T 1, s), MTV, mean diffusivity (diffusivity) and fractional anisotropy (FA) for 24 fascicles (tracts) based on cross-sectional measurements of 102 participants between the ages of 7 and 85 years. Each MRI parameter is sensitive to different tissue properties, and we use these measurements to examine biological principles of development and aging. We begin by focusing on R 1 changes over this 80-year period of the lifespan and then compare the R 1 measurements to the MTV, diffusivity and FA measurements. The R 1 value is affected first by the amount of tissue (macromolecules and lipid membranes) in a voxel: A voxel that is filled primarily with water will have a much smaller R 1 value (longer T 1) than a voxel that includes tissue. Second, the R 1 value is affected by the type of tissue [28] , [29] , [32] , [33] . Myelin, for example, has a particularly strong impact on R 1 values [27] for two reasons. First, it is a particularly dense tissue, in the sense that there are more macromolecules and fewer water molecules in a volume filled with myelinated axons compared with a volume filled with cellular tissue [34] . Second, myelin membrane has a high cholesterol and galactocerebroside content [35] . These molecules facilitate the longitudinal relaxation of water protons [32] , [36] . There were significant changes in R 1, MTV, diffusivity and FA between childhood, adulthood and old age for all fascicles. The time-course of the changes varied among fascicles and among MRI parameters. The diffusivity and FA measurements replicate previous observations [13] , and the R 1 and MTV measurements provide novel insight into the biological principles of white-matter development and aging. Fascicles vary substantially in terms of their amount of lifespan R 1 change. 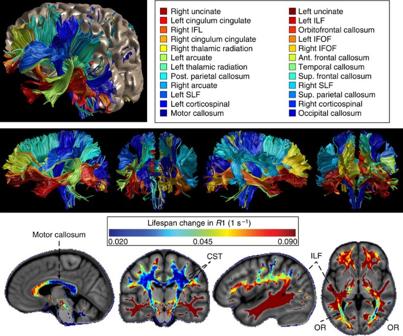Figure 1: Fascicles vary in the amount of lifespanR1 change. Twenty-four fascicles identified with the Automated Fibre Quantification software (AFQ) are shown for a 37-year-old male. In the top panel, the lateral aspect of the left hemisphere has been removed to view the white matter within the brain volume. In the middle panel, the white-matter fascicles are shown without the cortical surface. Each fascicle is coloured based on the amount of change inR1 (R1 at peak minusR1 at age 8) over the lifespan (cross-sectional); blue corresponds to less change and red to more change. The same fascicle colours are used throughout the manuscript. The bottom panel shows the magnitude ofR1 change for each voxel in the brain (computed by registering each participant’sR1 map to a customR1 template). The sharp differences between the development rates of adjacent tracts are clearly apparent in the corpus callosum (anterior versus posterior) and temporo-occipito white matter (ILF/IFOF versus optic radiations (OR)). Ant, anterior; Post, posterior; Sup, superior. Figure 1 shows each fascicle, color-coded based on the amount of R 1 lifespan change that can be modelled as a function of age (measured cross-sectionally). Some fascicles, such as the inferior longitudinal fasciculus (ILF), show substantial age-related change in tissue composition as indexed by R 1, while other fascicles, such as the corticospinal tract (CST) show more stable R 1 values over the lifespan. Figure 1: Fascicles vary in the amount of lifespan R 1 change. Twenty-four fascicles identified with the Automated Fibre Quantification software (AFQ) are shown for a 37-year-old male. In the top panel, the lateral aspect of the left hemisphere has been removed to view the white matter within the brain volume. In the middle panel, the white-matter fascicles are shown without the cortical surface. Each fascicle is coloured based on the amount of change in R 1 ( R 1 at peak minus R 1 at age 8) over the lifespan (cross-sectional); blue corresponds to less change and red to more change. The same fascicle colours are used throughout the manuscript. The bottom panel shows the magnitude of R 1 change for each voxel in the brain (computed by registering each participant’s R 1 map to a custom R 1 template). The sharp differences between the development rates of adjacent tracts are clearly apparent in the corpus callosum (anterior versus posterior) and temporo-occipito white matter (ILF/IFOF versus optic radiations (OR)). Ant, anterior; Post, posterior; Sup, superior. Full size image The uniqueness of each fascicle’s R 1 time-course can be appreciated by examining voxel-wise estimates of R 1 change. There are sharp changes in development rates at the border of fascicles. For example, R 1 in the optic radiation is stable over the lifespan (blue), while the immediately adjacent ILF and inferior fronto-occipital fasciculus change substantially (red). Even directly adjacent fibre tracts with different cortical destinations show very different developmental patterns. For example, within the corpus callosum the motor fibres (blue) are stable, while fibres destined for the prefrontal cortex change considerably (yellow-red). R 1 development and aging are symmetric for each fascicle We find that each tract has a signature R 1 value that is consistent along its length for a subject ( Supplementary Fig. 1 ). While the R 1 value along a tract is nearly constant, the mean R 1 value of a tract often differs substantially from the R 1 values of neighbouring tracts in the same hemisphere (>10 s.e.m., P <0.0001). From childhood (7 years of age) to adulthood (~40 years of age), R 1 increases significantly within all tracts, and the magnitude of change varies significantly among tracts ( Fig. 2 ). R 1 values for each tract reach their peak, mature level between 30 and 50 years of age. The values then decline, returning to their 8-year-old levels between age 70 and 80. For every tract we evaluated, the R 1 growth curves are well fit by a symmetric curve such as a second order polynomial (parabola) over the measured 80-year period of the lifespan. This implies that the rate of growth and decline are symmetric during a period of the lifespan lasting from the beginning of elementary school through senescence. As R 1 is sensitive to the creation of new tissue, particularly myelin [27] , the R 1 data are consistent with the idea that the rate of tissue loss during brain aging mirrors the rate of tissue creation between childhood and early adulthood. 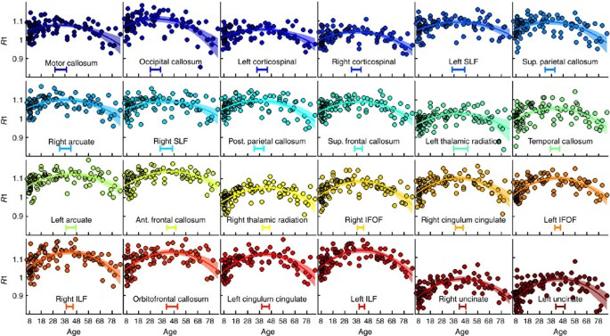Figure 2:R1 lifespan curves demonstrating each fascicle’s pattern of maturation and degeneration. R1 lifespan curves are shown for each of the 24 fascicles, ordered based on the amount of change inR1 over the lifespan. The width of the line denotes the 95% confidence interval around the second order polynomial model fit. There is a highly significant developmental increase and aging decline inR1 values for all fascicles. The age of peakR1 (±95% confidence interval) is shown by a bar at the bottom of each plot. TheR1 values for each individual do not depend on the specific dMRI acquisition used to define the tracts:R1 values are highly consistent when an individual’s tracts are defined using a lowb-value (1,000 m s−2) or highb-value (2,000 m s−2) acquision (R2=0.93). Post, posterior; Sup, superior. Figure 2: R 1 lifespan curves demonstrating each fascicle’s pattern of maturation and degeneration. R 1 lifespan curves are shown for each of the 24 fascicles, ordered based on the amount of change in R 1 over the lifespan. The width of the line denotes the 95% confidence interval around the second order polynomial model fit. There is a highly significant developmental increase and aging decline in R 1 values for all fascicles. The age of peak R 1 (±95% confidence interval) is shown by a bar at the bottom of each plot. The R 1 values for each individual do not depend on the specific dMRI acquisition used to define the tracts: R 1 values are highly consistent when an individual’s tracts are defined using a low b -value (1,000 m s −2 ) or high b -value (2,000 m s −2 ) acquision ( R 2 =0.93). Post, posterior; Sup, superior. Full size image Tracts differ substantially both in their mature R 1 values as well as the magnitude of R 1 changes over the lifespan. For example, the mature R 1 values of the anterior thalamic radiations and CST are equivalent to the childhood/old-age R 1 values of the cingulum, arcuate fasciculus, superior longitudinal fasciculus (SLF) and ILF. Moreover, the developmental increase and age-related decline in R 1 for the cingulum and ILF are nearly double that of the CST and anterior thalamic radiations. The uncinate fasciculus has a substantially lower R 1 value than all other tracts yet also shows a particularly large increase in R 1 during development and decline in R 1 during aging. Fascicles differ in the axon calibre distribution, myelination and packing density, and these properties influence information transmission and cortical computation [37] , [38] . Variations in mature R 1 levels and rate of change between fascicles reflect differences in the tissue composition. Changes in MTV predict changes in R 1 To better understand the biological underpinnings of the R 1 signal we model the relationship between developmental changes in R 1 and changes in macromolecule volume within each fascicle. Maps of MTV fraction were computed for each subject using a revised version of the method described in the study by Mezer et al . [7] It has been suggested that in brain tissue, R 1 is principally sensitive to the volume fraction of tissue (macromolecules and lipid membranes) versus water filling the voxel [6] , [7] , [33] . Creation of new non-water tissue (that is, MTV) within a voxel should cause a predictable increase in the voxel’s R 1. The amount of R 1 development was calculated for each fascicle as the difference in R 1 at 10 years of age versus adulthood (peak R 1 between 40 and 50 years of age). To test the relationship between R 1 changes and MTV changes we used a model [7] , [27] , [33] to predict the amount of MTV change for each fascicle based on the measurements of R 1 change: The measurements of MTV change closely matched the R 1-based predictions of MTV change ( R 2 =0.90), confirming that over development, new tissue is the principle mechanism underlying changes in R 1 ( Fig. 3 ). 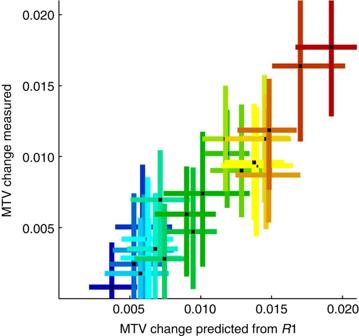Figure 3:R1 changes are principally driven by the creation of new tissue during development. MTV developmental change can be predicted based on theR1 measurements (x-axis) and this prediction closely matches the MTV measured changes (y-axis). Each point shows the magnitude of change (±1 s.e.) between age 10 and maturity (peak) for each fascicle (fascicle colours correspond toFigs 1and2). Figure 3: R 1 changes are principally driven by the creation of new tissue during development. MTV developmental change can be predicted based on the R 1 measurements ( x -axis) and this prediction closely matches the MTV measured changes ( y -axis). Each point shows the magnitude of change (±1 s.e.) between age 10 and maturity (peak) for each fascicle (fascicle colours correspond to Figs 1 and 2 ). Full size image Diffusivity changes more in development than in aging Replicating previous reports, mean diffusivity declines rapidly between childhood and adulthood, but then shows a slow and steady increase beginning in the late 30s and 40s (ref. 13 ; Supplementary Fig. 2 ). The diffusivity data are not well fit by a symmetric model such as a second order polynomial because the rate of change in development is much more rapid than the change in aging. A Poisson curve captures this asymmetry [13] . Unlike R 1 values, diffusivity values at age 80 do not return to their 8-year-old level. Diffusivity development rates also vary among tracts. For example, the SLF and cingulum show significantly more lifespan change than the CST. This observation is consistent with previous reports [13] . Within each tract the diffusivity and R 1 lifespan curves differ substantially from each other ( Fig. 4a ). Hence, these two parameters measure different biological processes in the white-matter. There is only a weak relationship between the amount of change in R 1 and diffusivity for a tract ( r =0.39, P =0.06). For example, the R 1 values in the ILF change considerably more (150%) than the R 1 values in the SLF. Yet, there is no difference in their lifespan diffusivity changes. In a separate example, diffusivity in the left SLF changes much more (50%) than in the left CST. Yet there is no difference in their lifespan R 1 changes. 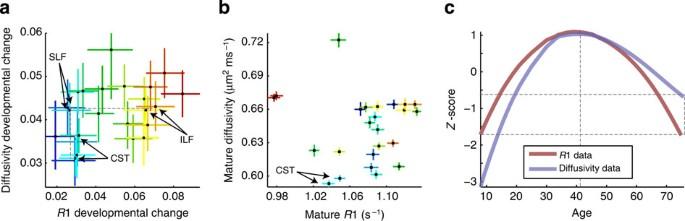Figure 4: Developmental processes drivingR1 and diffusivity development are independent. (a) Each point shows the magnitude ofR1 and diffusivity change during development. TheR1 changes are not well-predicted by the diffusivity change. For example, the inferior ILF shows significantly moreR1 change than the SLF (P<0.01) but they show the same amount of diffusivity change. (b) A tract’s matureR1 value is not well-predicted by its mature diffusivity value. This observation highlights that each measure is sensitive to different properties of the tissue. Each point shows a tract’s mean (± 1 s.e.)R1 and diffusivity value during adulthood. (c)R1 and diffusivity curves were standardized (z score, y-axises) and plotted on the same normalized axis to show the similarities and differences between these measures over the lifespan x-axis (the diffusivity curve was also inverted to make comparison easier). Diffusivity grows more rapidly and declines more slowly thanR1. The diffusivity lifespan curve is asymmetric for every fascicle and for each fascicle the shape of the diffusivity lifespan curve differs systematically from theR1 lifespan curve. BothR1 and diffusivity peak around the same age. Figure 4: Developmental processes driving R 1 and diffusivity development are independent. ( a ) Each point shows the magnitude of R 1 and diffusivity change during development. The R 1 changes are not well-predicted by the diffusivity change. For example, the inferior ILF shows significantly more R 1 change than the SLF ( P <0.01) but they show the same amount of diffusivity change. ( b ) A tract’s mature R 1 value is not well-predicted by its mature diffusivity value. This observation highlights that each measure is sensitive to different properties of the tissue. Each point shows a tract’s mean (± 1 s.e.) R 1 and diffusivity value during adulthood. ( c ) R 1 and diffusivity curves were standardized (z score, y-axises) and plotted on the same normalized axis to show the similarities and differences between these measures over the lifespan x-axis (the diffusivity curve was also inverted to make comparison easier). Diffusivity grows more rapidly and declines more slowly than R 1. The diffusivity lifespan curve is asymmetric for every fascicle and for each fascicle the shape of the diffusivity lifespan curve differs systematically from the R 1 lifespan curve. Both R 1 and diffusivity peak around the same age. Full size image Furthermore a tract’s mature diffusivity level is not well-predicted by its mature R 1 level. For example, at maturity the CST has the lowest diffusivity value of all the tracts yet its mature R 1 level is not comparatively high or low ( Fig. 4b ). Hence the two measurements capture different properties of the underline tissue like axons and glia that compose a fascicle. Multiple processes govern white-matter development and aging Two observations support the assertion that there are multiple, independent, biological processes governing age-related changes in white-matter tissue properties and that qMRI is sensitive to these processes. First, the amount of change in R 1 is independent of the amount of change in diffusivity. A large change in R 1-sensitive tissue is not linked to a large change in diffusivity-sensitive tissue ( Fig. 4a ). Second, the two measures follow different lifespan functions (Parabola versus Poisson; Fig. 4c ). To understand the extent of the relationship between R 1 and diffusivity, we used a polynomial model to predict R 1 from diffusivity for each tract. On an average, diffusivity predicts 25% of the variance in R 1 values (95% confidence interval (CI)=19–30%). Consider the residual errors in this model (that is, the variance in R 1 that is not predicted by diffusivity or Δ R 1). If lifespan changes in R 1 and diffusivity arise from the same biological processes, there should be no relationship between Δ R 1 and age. But in fact, age predicts a significant amount (on an average 10%) of the Δ R 1 variation ( P <0.01, 95% CI=8–12% variance explained). This highlights (1) that each parameter is weighted to be sensitive to different properties of the tissue, and (2) different tissue properties evolve independently over the lifespan. There are similarities between the measures, but knowing the amount and timing of change in diffusivity for a tract only weakly predicts the change in R 1 ( Fig. 4a ). The similarities and differences between R 1 and diffusivity can be appreciated by plotting the mean lifespan curve for each parameter on the same graph ( Fig. 4c ). The measurements for all 24 fascicles are summarized with a local regression model. The local regression model can assume any smooth shape and is a non-parametric way to compare the shape of lifespan curves for different parameters. Interestingly both curves develop until they peak at an age of 33 years, remain stable for ~10 years, and then reverse their direction with aging. However the rate of diffusivity growth is steeper than the rate of R 1 growth, while the rate of diffusivity decline is shallower. While R 1 shows a symmetric shape, with an equivalent value in childhood and senescence, diffusivity values do not return to their childhood levels. The difference in the preferred models for the different qMRI measures supports the hypothesis that multiple active biological processes drive changes in the white matter. Less lifespan change in FA compared with R 1 or diffusivity The R 1 and diffusivity values changed substantially and systematically over the lifespan: 25–45% of the variation in the measurements for a tract is predicted as a function of age. Over the lifespan, mean tract FA changes are smaller, and on an average only 10% of the variation in FA values across subjects are accounted for by age (for any model in either the b =2,000 or the b =1,000 data sets). FA values are highly influenced by the distribution of axon orientations within a voxel (coherence) [25] , [26] , [39] , and this feature of the white matter may be stable across the ages we measured. There is a lot of variability of the FA along each tract, and this variation is far larger than the age-related FA changes ( Supplementary Fig. 1 ). The observed FA variation along each tract was equivalent for the low and high b -value data sets. Hence, tracts do not have a signature FA value that is consistent along the tract length [39] . Analyses of FA development should model the biological processes driving FA change at specific locations along the tract. Evaluation of retrogenesis The principle of retrogenesis is widely discussed in the literature [18] , [19] , [20] , [21] , but it has not been formalized into a mathematical model and evaluated with respect to lifespan measurements. Hence there are multiple, dissociable, hypotheses that are consistent with the principle of retrogenesis. The ‘gain-predicts-loss’ hypothesis proposes that the rate of change is mirror-symmetric in development and aging: the more that is gained before the peak, the more that will be lost after the peak. The ‘last-in-first-out’ hypothesis states that the last regions to develop are the first to decline. This hypothesis predicts that the age at which development ends is negatively correlated with the age at which degeneration begins: Early development predicts a long period of stability and a late decline. These two ideas are related, however the gain-loss prediction is about the symmetry of the curve on either side of maturity, and the last-in-first-out prediction concerns the relative timing of a region reaching its mature state and the region beginning to degenerate. To quantitatively evaluate the fit of these lifespan hypotheses to white matter changes between the ages of 7 and 85, we fit the measurements from each tract to four different models (see Methods and Supplementary Fig. 3 ). One model is a simple parabola (second order polynomial) that captures the idea of gain-predicts-loss. The second model comprises multiple linear segments joined at hinges (piecewise linear); this model tests the hypothesis that the timing of development and decline are correlated (last-in-first-out). The third model is a Poisson curve that, in contrast to the parabola, has an asymmetric rise and decline. Finally, a local regression model makes no assumptions about the lifespan data and serves to capture any systematic deviations of the data from the model predictions. We evaluate the accuracy of each model using leave-one-out cross validation. Cross-validated estimates of model accuracy ( R 2 ) will decrease when an unnecessary parameter is included in a model (over fitting). Hence, the cross-validated estimates of R 2 can compare the accuracy of these different models. Consistency of R 1 with the gain-predicts-loss hypothesis We tested the gain-predicts-loss hypothesis by fitting a second order polynomial (parabola) to the lifespan measurements ( Fig. 5a ). The parabola fit the R 1 data for each tract as well or better than the more complex models (median R 2 =24%). Each tract matures at the same rate that it declines and a tract’s R 1 values are identical when measured at symmetric ages around the peak of the curve ( Fig. 5b,c ). 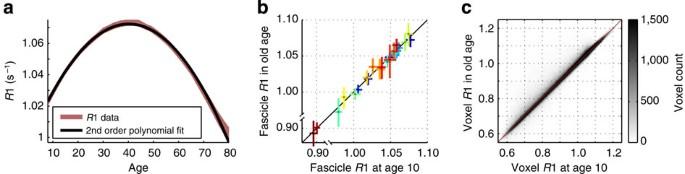Figure 5:R1 maturation and degeneration have symmetric slopes. (a) Mean lifespanR1 curve (red) combining the data from all tracts is superimposed on the prediction of the second order polynomial model (black). The mean curve was calculated by fitting a local regression model to the data for all the tracts; the width of the coloured line corresponds to the s.e. of the model. ForR1, there is no systematic difference between the data and the prediction of the symmetric parabola. For every age, the model prediction is within 1 s.e. of the measurement (diffusivity shown inSupplementary Fig. 4). (b) The symmetry of change inR1 over the lifespan can be appreciated by plotting theR1 value in childhood and senescence for each individual tract. The age of peakR1 was calculated and values are plotted at age 10 and at a symmetric number of years past the peak (senescence). In senescence,R1 values return to the same level they were in childhood. For diffusivity, the values do not return to their childhood level (Supplementary Fig. 4b). (c)R1 changes over the lifespan are symmetric for most voxels in the brain. Each participant’sR1 map was aligned to a custom,R1 template and the voxelR1 value was calculated at age 10 and a symmetric number of years past that voxel’s peak. The childhood and old-ageR1 values are closely matched for each white-matter voxel (R2=0.70). Figure 5: R 1 maturation and degeneration have symmetric slopes. ( a ) Mean lifespan R 1 curve (red) combining the data from all tracts is superimposed on the prediction of the second order polynomial model (black). The mean curve was calculated by fitting a local regression model to the data for all the tracts; the width of the coloured line corresponds to the s.e. of the model. For R 1, there is no systematic difference between the data and the prediction of the symmetric parabola. For every age, the model prediction is within 1 s.e. of the measurement (diffusivity shown in Supplementary Fig. 4 ). ( b ) The symmetry of change in R 1 over the lifespan can be appreciated by plotting the R 1 value in childhood and senescence for each individual tract. The age of peak R 1 was calculated and values are plotted at age 10 and at a symmetric number of years past the peak (senescence). In senescence, R 1 values return to the same level they were in childhood. For diffusivity, the values do not return to their childhood level ( Supplementary Fig. 4b ). ( c ) R 1 changes over the lifespan are symmetric for most voxels in the brain. Each participant’s R 1 map was aligned to a custom, R 1 template and the voxel R 1 value was calculated at age 10 and a symmetric number of years past that voxel’s peak. The childhood and old-age R 1 values are closely matched for each white-matter voxel ( R 2 =0.70). Full size image The additional flexibility in the piecewise linear model (median R 2 =23%) and local regression (median R 2 =23%) model are not useful for describing R 1 over the measured 80 years of the lifespan because the rate of rise and decline in R 1 are equal. The additional flexibility in those models fits the noise (over-fits) and increases the cross-validated error. The R 1 curves are consistent with the ‘gain-predicts-loss’ principal of white-matter development and aging. Tracts with large R 1 gains during childhood show large R 1 declines during aging and tracts with minimal R 1 gains do not show substantial aging-related degeneration. Measured by R 1, the aging process (ages 50–85) resembles the development process in reverse (ages 7–50). Diffusivity shows differences between development and aging Measured by diffusivity, the aging process is not just the reverse of development. The R 1 data adheres to the prediction of the gain-predicts-loss model, but the diffusivity data does not. The slope of diffusivity development is significantly steeper than the slope of aging ( P <0.001, tested with the piecewise linear model) and a parabola is unable to capture the asymmetry of diffusivity change on either side of the peak ( Supplementary Fig. 4 ). A Poisson curve captures the asymmetric change [13] and fits the diffusivity measurements better than all other models ( P <0.001, median R 2 =42%). For diffusivity the local regression and piecewise linear models also fit the measurements better than the parabola ( P <0.001), but not as well as the Poisson curve ( P <0.001). Unlike R 1, the rate of change of diffusivity differs between development and aging. Last-in-first-out hypothesis doesn’t predict R 1 or diffusion The data do not support the last-in-first-out hypothesis: the age at which a tract reaches maturity does not predict the age at which it begins to decline. 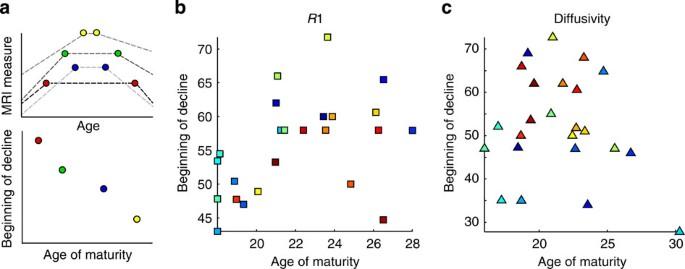Figure 6: The last-in-first-out hypothesis does not match theR1 or diffusivity measurements. The last-in-first-out hypothesis predicts that fascicles which reach maturity later begin declining earlier. A piecewise linear model independently fits the slope and timing of maturation and aging and can test this hypothesis. (a) The left panel shows a series of hypothetical piecewise linear models that are consistent with the last-in-first-out hypothesis. In each hypothetical tract lifespan curve, the age that the MRI parameter reaches its mature value is negatively correlated with the age it begins to decline. (b,c) The right two panels show the age of maturity (x-axis) plotted against age of decline (y-axis) as determined from the piecewise linear model of (b)R1 and (c) diffusivity measurements. The data are not consistent with the last-in-first-out hypothesis: There is no systematic relationship between the age at which a tract matures and the age at which it begins to decline. Figure 6 shows a scatter plot of the two transition point parameters of the three segment, piecewise linear model. The last-in-first-out hypothesis predicts a negative correlation between these two parameters such that earlier maturation predicts later aging. For R 1, there was a weak positive correlation ( r =0.43, P =0.04), which is contrary to the prediction of the last-in-first-out hypothesis. There is no significant correlation for diffusivity ( r =−0.18, P =0.38) or FA ( r =−0.13, P =0.52). If there is a link between the time a tract reaches maturity and the time it begins to decline, the effect is small. Figure 6: The last-in-first-out hypothesis does not match the R 1 or diffusivity measurements. The last-in-first-out hypothesis predicts that fascicles which reach maturity later begin declining earlier. A piecewise linear model independently fits the slope and timing of maturation and aging and can test this hypothesis. ( a ) The left panel shows a series of hypothetical piecewise linear models that are consistent with the last-in-first-out hypothesis. In each hypothetical tract lifespan curve, the age that the MRI parameter reaches its mature value is negatively correlated with the age it begins to decline. ( b , c ) The right two panels show the age of maturity ( x -axis) plotted against age of decline ( y -axis) as determined from the piecewise linear model of ( b ) R 1 and ( c ) diffusivity measurements. The data are not consistent with the last-in-first-out hypothesis: There is no systematic relationship between the age at which a tract matures and the age at which it begins to decline. Full size image From quantitative models to individual diagnosis R 1 is a quantitative measure of tissue at a given magnetic field strength (for example, 3T) meaning that R 1 values are independent of the specific scanner hardware [7] , [31] , [40] . Hence, a model of R 1 growth and decline can be used as norms for clinical and scientific comparisons across institutions. To confirm that our R 1 measurements are truly quantitative and do not depend on the specific hardware that is used to measure the brain, we performed three control experiments. First, we compare fascicle R 1 values for the same individual measured in separate sessions with two different head coils (a custom made Nova 32-channel coil versus a stock GE 8-channel coil) and find that the R 1 values are highly stable ( Fig. 7a , R 2 =0.95). Second, we compare R 1 measurements acquired at 1 mm 3 resolution on a GE 3T scanner at the Stanford University versus R 1 measurements for the same individual measured at 2 mm 3 on a Siemens 3T scanner at the Jerusalem University. The Siemens measurements are noisier because the sequence was optimized for the GE scanner: this can be improved. But importantly, even with the differences in pulse sequences, there was no systematic difference between the two measurements (that is, bias) ( Fig. 7b , R 2 =0.79). Finally we quantify the robustness of the measurements to head motion by measuring the same individual twice on the same scanner, first, with minimal head motion and second, with moderate head motion. The moderate head motion caused characteristic artifacts in the raw images (for example, ripples) but did not induce any systematic bias to the R 1 measurements ( Fig. 7c , R 2 =0.98). 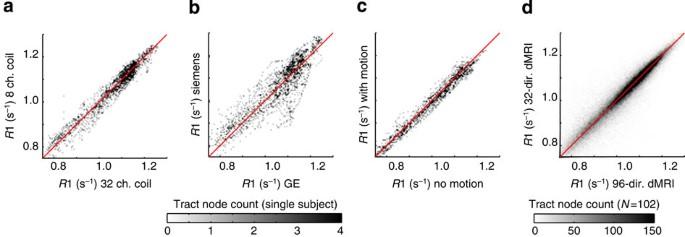Figure 7:R1 measurements are reliable across differences in scanner hardware and head movements. (a)R1 values sampled along the length of the 24 fibre tracts within an individual scanned using two different head coils, (b) two scanner vendors (GE versus Siemens) and (c) minimal versus moderate head motion. (d)R1 values sampled along fiber tracts estimated from a 96-direction,b=2,000 dMRI acquisition and a 30-direction,b=1,000 dMRI acquisition (N=102). AFQ reliably estimates the same fibres in both acquisitions, and the fascicleR1 values are consistent. Figure 7: R 1 measurements are reliable across differences in scanner hardware and head movements. ( a ) R 1 values sampled along the length of the 24 fibre tracts within an individual scanned using two different head coils, ( b ) two scanner vendors (GE versus Siemens) and ( c ) minimal versus moderate head motion. ( d ) R 1 values sampled along fiber tracts estimated from a 96-direction, b =2,000 dMRI acquisition and a 30-direction, b =1,000 dMRI acquisition ( N =102). AFQ reliably estimates the same fibres in both acquisitions, and the fascicle R 1 values are consistent. Full size image The stability of the R 1 measurements across different hardware, pulse sequence, image resolution and subject motion, mean that the normative model of healthy R 1 development can be used to detect and quantify tissue loss in individual patients with degenerative diseases of the white matter including MS ( Fig. 8 ). Each individual with MS ( N =10) has regions of the white matter that are substantially different from the model prediction (>3 s.d.). These highly abnormal regions correspond to MS lesions. To test the specificity of this approach, a group of healthy, age-matched participants was held out of the model construction and compared with the normative model. The healthy participants did not have regions of highly abnormal R 1 values ( Fig. 8c , black curve). The median R 1 value across all white-matter voxels for each individual with MS is also below the mean for his or her age ( Fig. 8c , blue tick marks); this effect is significant for the group ( P <0.001). 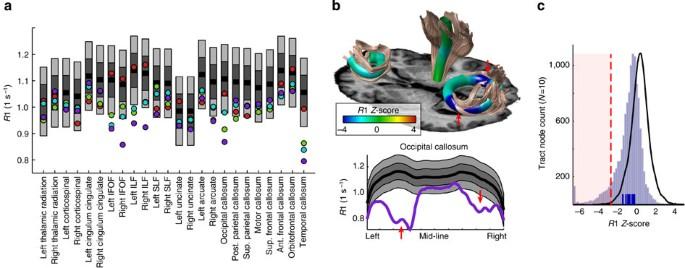Figure 8: Automated diagnosis and quantification of white-matter lesions based onR1 lifespan curves. (a) Four patients with multiple sclerosis (43–45 years of age) are compared with age-matched norms based on the model ofR1 development (SeeFig. 2). The grey bands show 1 and 2 s.d. intervals around the mean for 44-year-olds on each tract. The meanR1 values for tracts with demyelinating MS lesions are substantially below the healthyR1 values (>3 s.d.) but even the normal appearing white matter has slighly lowerR1 values than the average. (b) Comparing individual patient data with a group localizes lesions and quantifies tissue loss. The tracts are shown for one patient (purple), who has large lesions in occipital callosal fibres in both hemispheres. (c) A simple threshold identifies locations with substantial tissue loss. Ten age-matched, control subjects were left out of the curve-fitting procedure and for each location on the tracts we compared theR1 value with the norm for the relevant position (black line). For the healthy controls, very few locations on any tract exceed a 3-s.d. threshold, highlighting the specificity of theR1 comparison. The same analysis was applied to the MS patients (N=10, light blue histogram). These patients have many locations, whereR1 values are more than 3 s.d. below the age-matched norms. Each patient’s medianR1 white-matter value (blue tick marks) is also below the norms. Figure 8: Automated diagnosis and quantification of white-matter lesions based on R 1 lifespan curves. ( a ) Four patients with multiple sclerosis (43–45 years of age) are compared with age-matched norms based on the model of R 1 development (See Fig. 2 ). The grey bands show 1 and 2 s.d. intervals around the mean for 44-year-olds on each tract. The mean R 1 values for tracts with demyelinating MS lesions are substantially below the healthy R 1 values (>3 s.d.) but even the normal appearing white matter has slighly lower R 1 values than the average. ( b ) Comparing individual patient data with a group localizes lesions and quantifies tissue loss. The tracts are shown for one patient (purple), who has large lesions in occipital callosal fibres in both hemispheres. ( c ) A simple threshold identifies locations with substantial tissue loss. Ten age-matched, control subjects were left out of the curve-fitting procedure and for each location on the tracts we compared the R 1 value with the norm for the relevant position (black line). For the healthy controls, very few locations on any tract exceed a 3-s.d. threshold, highlighting the specificity of the R 1 comparison. The same analysis was applied to the MS patients ( N =10, light blue histogram). These patients have many locations, where R 1 values are more than 3 s.d. below the age-matched norms. Each patient’s median R 1 white-matter value (blue tick marks) is also below the norms. Full size image We combined qMRI measurements of R 1 and MTV with dMRI and tractography to model white matter development and aging over an 80-year period of the lifespan. Developmental processes create new tissue that displaces water, leading to higher R 1, MTV and FA and lower diffusivity within the white matter. The R 1 decline with aging is mirror-symmetric with the R 1 increase during development. We confirm that for each fascicle, R 1 changes in development are tightly coupled to changes in MTV. In the white matter, a majority of the macromolecules are contained in myelin membrane [34] . The symmetry of the R 1 changes during development and aging might be explained if the tissue created late in childhood is equal to the tissue lost during aging. Unlike R 1, the diffusivity change during aging is substantially slower than the diffusivity change during childhood. Even though tissue is lost during aging, the elderly brain does not revert back to the biology of a child’s brain. There are multiple active lifespan processes and not all of them are symmetric. This observation is supported by histology in aging macaques, showing that axons and myelin are lost but the continued creation of new astrocytes, microglia and oligodendrocytes fill the empty space [41] , [42] . We used the qMRI measurements to test three quantitative hypotheses regarding the biological principles of white-matter development and aging. Evidence supports the gain-predicts-loss ( Fig. 5 ) and multiple-biological-process hypotheses ( Fig. 4 ), but the lifespan curves for R 1, diffusivity and FA contradict the last-in-first-out hypothesis ( Fig. 6 ). These models concern changes in brain tissue as the brain approaches maturity and begins to decline, and there are certainly additional processes that drive in utero [43] and infant white-matter development [5] . The rapid changes that occur in utero and during infant development might be discontinuous with the changes measured between childhood and 85 years of age. By extending the measured age range, future work can confirm whether the symmetry of the curves extends from infancy through the end of life or if additional, independent mechanisms drive white-matter changes at the beginning and end of life. These observations highlight two important points. First, it is unlikely that a single model characterizes changes in the myriad of cell types in the brain. There is value, then, in using multiple qMRI measurements that are sensitive to different tissue properties. Second, formalizing ideas such as ‘retrogensis’ into a computational framework is essential for determining whether it is a suitable principle to characterize brain development. The concept of retrogensis formalized as a symmetric curve accurately predicts changes in R 1 over the lifespan, while retrogensis formalized under the last-in-first-out model does not fit the data. A major goal of human neuroscience is to understand the cellular processes in the living human brain that drive changes in cognitive function over the lifespan. There is an extensive literature linking the biophysics of macromolecules composing brain tissue to MR properties such as R 1, MTV and diffusivity. These qMRI measurements offer a unique opportunity to bridge the gap between cognitive, systems and cellular neuroscience. Before discussing how qMRI measurements extend our understanding of the neurobiology of development and aging, it is useful to consider what is already known from invasive studies employing animal models and post mortem histology. Beginning in the late prenatal period and continuing through childhood and young adulthood, axons grow in calibre and oligodendrocytes wrap myelin around these axons [44] . With each additional wrap of myelin, the outer diameter of the axon increases. This additional tissue provides a barrier to the diffusion process and reduces the overall water content of the tract (which also affects R 1) as macromolecules fill the space that was once occupied by water molecules. Even though a substantial number of underused axons are removed (pruning) during development to free space for the growth of pertinent axons [45] , [46] , overall there is an increase in macromolecule content and a decrease in water content as a child’s brain approaches maturity [47] . The myelination process is determined both by intrinsic genetic codes and extrinsic environmental factors [44] , [48] . The level of electrical activity of an axon influences myelination, meaning that the myelination process is modified through experience [48] , [49] . Myelination speeds signal conduction between distant cortical regions and together the distribution of myelin and axon calibre in a pathway determines the rate, quantity and nature of signals that a pathway transmits [37] , [38] , [50] . There is a period of relative stability before the white matter once again undergoes substantial changes due to aging processes. Even though the number of neurons in the cortex remains relatively constant, axons in the white matter begin to degenerate [51] . Sandell and Peters [41] demonstrate that the packing density of axons in the macaque optic nerve declines from an average of 28.85 per 100 μm 2 in mature monkeys to 17.18 per 100 μm 2 in old monkeys. The degeneration of axons appears to be coupled with degeneration of their myelin sheaths: there is as much as a fivefold increase in the number of microglia in aging fascicles and many microglia are engorged with phagocytosed myelin. Beyond the increase in the numbers of microglia, new oligodendrocytes develop from oligodendrocyte progenitor cells and the fanning astrocyte processes expand to fill many gaps left by the degenerating axons [42] . As the brain ages, some tissue degenerates but new tissue is also created leading to large-scale changes in the cellular composition of the white matter. The different mechanisms present in development and aging are reflected in the quantitative MR data. There is a rapid change in R 1 and diffusivity during development, with a symmetric rapid decline in R 1 over aging but slow, gradual change in diffusivity. One hypothesis that explains the pattern of results is this: glial tissue that is created in the aging brain has a substantially lower R 1 value than the myelinated axons that are lost. Diffusivity changes less because glial membrane barriers effectively restrict water movement. Glial proliferation in the aging brain could explain why diffusivity does not decline as sharply as R 1. Myelin membrane is particularly rich in cholesterol and galactocerebroside [35] , [47] . These two macromolecules have a particularly large impact on R 1 relaxation rates of water molecules [32] . Moreover, unlike other cell structure, myelin has many tightly wrapped membrane layers yielding particularly high density of macromolecules versus water molecules. R 1 decreases roughly linearly with the volume of water molecules in a voxel [7] , [52] , [53] . The lifespan data demonstrate that R 1 changes can explain with great accuracy the MTV changes. Many studies suggest that R 1 is a good index of myelin variation across brain regions [27] , [54] , [55] , [56] ; however, any decrease in water content due to additional tissue in a voxel also increases R 1. Moreover, biochemical processes that change the type of macromolecules and ions affect R 1 without affecting the MTV values. For this reason, both measurements contribute to our understanding of white-matter maturation and degeneration. R 1 and diffusivity measurements differ substantially when comparing voxels packed with cells (grey matter) and those packed with myelinated axons (white matter). The diffusivity in grey and white matter is roughly equivalent, suggesting that diffusion barriers are similar in both types of tissue. But the mean R 1 in white matter is almost double the mean R 1 in grey matter [7] , [57] . In aging, R 1 declines steeply but diffusivity only slowly. Hence, the data support the view that in aging there is degeneration of myelinated white-matter axons and proliferation of glia. What might cause the symmetry of the R 1 lifespan curves? The link between R 1 growth and R 1 decline may reflect a general phenomenon regarding the link between plasticity and vulnerability of a brain region. Connections between gene expression across the lifespan are an important future step for understanding the molecular mechanisms that produce the circuit level changes we measure in the living human brain. These data provide the first benchmark of R 1 in the healthy brain across a large portion of the lifespan. Because the R 1 data are quantitative, an individual scanned at any location in the world can be compared with the normative lifespan curves established in this study. We demonstrate the utility of these models for detection and quantification of MS lesions ( Fig. 8 ). This approach supports the goal of using qMRI to quantitatively monitor healthy development and aging or disease progression within an individual. While the current sample reported here is too small to characterize the normal variation in white-matter tissue properties across demographic groups, we hope that data sharing across institutions will assist in obtaining larger, more diverse samples. These data could prove useful in the early identification, treatment and post-treatment monitoring of myelin abnormalities in the developing, mature and aging brain. Additional measurements are needed to understand how changes in myelin affect cortical computations and resulting behaviours. Combining in vivo biological measurements with behavioural measurements will lead to models that explain the coupling between biological and cognitive development. DMRI has demonstrated robust correlations between diffusion properties and behaviour, driving an interest in the role of white matter in cognition but leaving the biology of these correlations a mystery [24] . Combining diffusion tractography with measures of diffusivity and R 1 is a step towards inferring the biological mechanisms that link white-matter tissue to cognition. Summary We used qMRI to measure changes in the tissue properties of 24 major white-matter fascicles over the lifespan. The protocol included (1) a high angular resolution diffusion imaging (HARDI) sequence that was optimized for the identification of each fascicle and the quantification of each fascicle’s diffusion properties and (2) a technique to quantitatively map R 1 (1/ T 1), the longitudinal relaxation rate of the MR signal, in each fascicle [7] . We measured 102 subjects between the ages of 7 and 85 years. The Automated Fibre Quantification (AFQ) software package was used to identify 24 major white-matter fascicles from each individual’s diffusion data and map the qMRI measurements to these fascicles [39] . The following sections describe the subjects, MRI protocol and data processing in detail. Example code and data is available at https://github.com/jyeatman/lifespan . Subjects The Stanford University Institutional Review Board approved all data collection procedures and each adult participant provided informed consent and each child participant assent with the consent provided by their parent/guardian. The participants in the study were healthy volunteers recruited from the San Francisco Bay Area based on flyers, advertisements in local papers and school newsletters. All participants were screened for neurological, psychiatric and cognitive disorders. However subjects were not screened for disorders that are likely to occur later in life (for example, hypertension). The age distribution of the sample purposefully included more subjects in the age bins that were expected to show the largest change in tissue properties and fewer subjects in the age bins that were expected to have stable tissue properties. There were 32 participants of age 7–12, 14 participants of age 13–18, 12 participants of age 19–29, 11 participants of age 30–39, 7 participants of age 40–49, 9 participants of age 50–59, 8 participants of age 60–69, 9 participants of age 70–85, forming a total of 102 participants (51 female participants). dMRI acquisition and preprocessing All dMRI data were collected on a General Electric Discovery 750 (General Electric Healthcare, Milwaukee, WI, USA) equipped with a 32-channel head coil (Nova Medical, Wilmington, MA, USA) at the Center for Cognitive and Neurobiological Imaging at Stanford University ( www.cni.stanford.edu ). dMRI data were acquired using dual-spin echo diffusion-weighted sequences with full brain coverage. Diffusion weighting gradients were applied at 96 non-collinear directions across the surface of a sphere as determined by the electro-static repulsion algorithm [58] . In all subjects, dMRI data were acquired at 2.0 mm 3 spatial resolution and diffusion gradient strength was set to b =2000, s mm −2 . We acquired eight non-diffusion-weighted b =0 images at the beginning of each measurement. A second, independent, dMRI data set was acquired on each subject using a low b -value ( b =1000, s mm −2 ) 30-direction acquisition. Subjects’ motion was corrected using a rigid body alignment algorithm. Diffusion gradients were adjusted to account for the rotation applied to the measurements during motion correction. The dual-spin echo sequence we used does not require performing eddy current correction because it has a relatively long delay between the RF excitation pulse and image acquisition. This allows sufficient time for the eddy currents to dephase. A tensor model was fit to each voxel’s data using the RESTORE algorithm, which is designed to remove outliers from the fitting procedure and minimize the effects of pulsatility and motion-related artifacts [59] . Preprocessing was implemented in MATLAB (MathWorks, Natwick, MI, USA) and are publically available as part of the vistasoft git repository ( http://github.com/vistalab/vistasoft/mrDiffusion ; see dtiInit.m). Quantitative T 1 mapping protocol R 1 relaxation was measured from spoiled gradient echo (spoiled-GE) images acquired at different flip angles (á=4°, 10°, 20°, 30°, TR=14 ms, TE=2.4 ms). The scan resolution was 1 mm 3 . In addition to the 102 subjects measured on a GE scanner, one subject was also measured on a 3T Siemens scanner in Jerusalem. The transmit-coil inhomogeneity was corrected by comparing with R 1 measured with an additional spin echo inversion recovery (SEIR) scan [7] that is free from transmit-coil inhomogeneity [7] , [60] . The SEIR was done with an echo planar imaging (EPI) read-out, a slab inversion pulse and spectral spatial fat suppression. For the SEIR-EPI acquisition the TR was 3 s; Echo time was set to minimum full; inversion times were 50, 400, 1,200, 2,400 ms. We used 2 mm 2 in-plane resolution with a slice thickness of 4 mm. The EPI read-out was performed using 2 × acceleration to minimize spatial distortions. We used the ANTS software package to register the spoiled-GE images to match the SEIR-EPI image [61] . The transmit-coil inhomogeneity was calculated by combining the un-biased SEIR R 1 fits with the spoiled-GE data [7] . We use the estimated transmit-coil inhomogeneity and the multi flip-angle spoiled-GE measurements to derive the R 1 maps. These were calculated using a nonlinear least-squares fitting procedure to minimize the difference between the data and the spoiled-GE signal equation predictions [62] . We release the R 1 analysis pipeline as open-source MATLAB code ( https://github.com/mezera/mrQ ). Quantification of white-matter tissue properties The AFQ software package was used to identify each fibre tract and quantify Tract Profiles of tissue properties along the tract trajectory [39] . There were a number of substantial additions and revisions to the AFQ software for the analyses reported here, and like previous versions we release AFQ (v1.1) as open-source MATLAB code ( https://github.com/jyeatman/AFQ ). The major updates to the code are described here with additional details in the on-line revision history. AFQ uses a three-step procedure to identify each of the 24 fibre tracts in an individual’s brain. First, a tractography algorithm estimates a whole-brain connectome of fibre tracts. Deterministic streamlines tracking based on a tensor model is the default algorithm [63] . Second, fibre tract segmentation is done with a two way-point region of interest (ROI) procedure, in which each fibre from the whole-brain connectome becomes a candidate for a specific fibre group if it passes through two ROIs that define the trajectory of the fibre group [64] . Third, fibre tract refinement is done by comparing each candidate fibre to a fibre tract probability map, and removing each candidate that passes through regions of the white matter that are unlikely to be part of the tract [65] . Finally, the tract is summarized by a curve that is at the central position of all the tract fibres. The curve is created by defining 100 sample points along each fibre and robustly computing the mean position of the corresponding sample points. The robust mean is computed by estimating the three-dimensional Gaussian covariance of the sample points and removing fibres that are more than 5 s.d. from the mean. AFQ (v1.1) includes an additional tract cleaning procedure in which fibres with aberrant cortical endpoints are removed from the fibre group. This is achieved by warping the cortical labels from the MNI-AAL atlas [66] to an individual’s native space, and making sure each fibre in the group starts and ends within 4 mm of its known cortical destination. This a priori knowledge of fibre endpoint is only imposed at a very course resolution as to not bias new discoveries that come with improved tractography algorithms (for example, the arcuate spans from the lateral temporal to the lateral frontal lobe and the uncinate spans from the anterior temporal to the frontal lobe). Finally, each fibre in the group is flipped such that all fibres start and end in the same cortical zone and span the same direction (for example, posterior to anterior). These revisions increase the accuracy of Tract Profiles that are calculated for the full trajectory of the fibre group, from the cortical start to the cortical termination, rather than confining the analysis to the portion of the tract spanning between the two defining ROIs. AFQ (v1.1) includes eight additional callosal fibre groups that were not included in the previous release: occipital, posterior parietal, superior parietal, motor, superior frontal, anterior frontal and orbitofrontal and temporal callosal projections. Two ROIs placed in homologous regions of each hemisphere are used to segment the eight callosal fibre groups (as described in ref. 67 ). The occipital and posterior parietal ROIs are drawn on the coronal plane at the intersection of the calcarine and parieto-occipital sulci. The boundary between these ROIs separate fibres destined for occipital and parietal cortices. The superior parietal, motor and superior frontal ROIs are drawn on the axial plane, superior to the corpus callosum, where the central sulcus has an omega (Ω) shape. The superior parietal ROI covers the posterior portion of this plane and goes as far anterior as the central sulcus. The motor ROI extends from the central sulcus to the precentral gyrus. The superior frontal ROI covers the anterior portion of the plane. The anterior frontal and orbitofrontal ROIs are drawn on the plane half way between the genu of the corpus callosum and the frontal pole. The orbitofrontal ROI covers the most inferior gyrus in this plane and the anterior frontal ROI covers the superior portion of this plane. The temporal ROI is draw in a coronal plane and covers the white matter adjacent to the posterior horn of the lateral ventricles know as the tapetum. For these eight callosal groups, the fibre tract refinement stage was not necessary. The anterior frontal and occipital callosal groups are highly overlapping with the forceps major and forceps minor fibre groups (included in AFQ v0.1). Hence, only the new callosal groups were used as in the current analysis making for 24 tracts in total. Tissue properties are calculated along the trajectory of the fibre group by first resampling each fibre to 100 equally spaced nodes and then interpolating the value from a coregistered qMRI image at each node along each fibre. The maps of scalar parameters from the dMRI data are already in register with the fibre tracts and do not require additional alignment. To coregister a subject’s quantitative R 1 map to their dMRI data, we used the ANTS software package to warp the R 1 map to match the non-diffusion-weighted, B0 image [61] . This warping procedure corrects differences in image rotation and translation as well as local stretching and compression of the dMRI data due to EPI distortions. EPI distortions were minimal due to the 2 × ASSET acceleration used for the readout of the diffusion-weighted images, but some regions of the white matter were misaligned by 2–4mm if a simple rigid body alignment was used. After applying the diffeomorphic warp, manual inspection of the aligned images confirmed that the registration was accurate within ~1 mm. Tract Profiles of each parameter are calculated as a weighted sum of each fibre’s value at a given node, where a fibre is weighted based on its Mahalanobis distance from the core of the tract. The result is a vector of 100 measurements of each MRI parameter sampled equidistantly along the trajectory of each fascicle. Tract Profiles can then be averaged to produce a single mean value for each tract or models can be fit at each point along the Tract Profile. Voxel-wise analysis of R 1 data In addition to the analysis of fibre-tract R 1 values, we also conducted a voxel-wise analysis of R 1 development and aging. ANTS was used to build a custom R 1 template from the collection of individual subject R 1 maps (see the ANTS buildtemplateparallel.sh script). Then each model was fit voxel wise to characterize regional white-matter development and aging. Model fitting We fit four classes of models to explain changes in tissue properties as a function of age ( Supplementary Fig. 3 ). Model accuracy was quantified using leave-one-out cross-validation: The model was fit to the data leaving out one subject’s data point and then the model was used to predict this left out data point. This procedure is repeated for each subject and the difference between the model predictions and the measurements were used to calculate an un-biased estimate of the coefficient of determination ( R 2 ) using the following equation: where n is the number of measurements, y is the vector of measurements and ý is the vector of model predictions. Model 1 was a second order polynomial (parabola) with the following equation: where y is the vector of measurements and each w i is a weight that is estimated using ordinary least-squares regression. Model 2 was a five-parameter piecewise linear model. The first two parameters are the intercept and slope of change over development. The third and fourth parameters are transition points, the first of which being the age when development ends and the next being the age at which aging begins. Maturity is defined as the time between the two transition points during which tissue properties remain relatively constant. The fifth parameter is the slope of change during aging. The piecewise linear model was fit using the Levenberg–Marquardt algorithm with a least-squares cost function. Due to local minimum, we did a grid search over starting parameters and the model with the lowest mean squared error was retained. Model 3 was a Poisson curve with asymmetric rise and decline as described in ref. 13 with the following equation: Where each w i is a parameter estimated using the Levenberg–Marquardt algorithm with a least-squares cost function. Model 4 was a local linear regression model in which each data point was predicted based on a linear fit that considered a local window of data centered on that point. The local regression model was fit using weighted least squares, where each data point’s contribution to the fit was weighted based on its distance to the center of the window. We used a tricubic weighting function and a bandwidth of 20 years. The local regression model can assume any smooth shape and imposes very few constraints on the shape of a tract’s lifespan curve. Parameter reliability was estimated with bootstrapping. Unless otherwise stated, the results throughout the paper use the median and bootstrapped CI around the median to represent the central tendency and error of each estimate. How to cite this article : Yeatman, J. D. et al . Lifespan maturation and degeneration of human brain white matter. Nat. Commun. 5:4932 doi: 10.1038/ncomms5932 (2014).